Overlap between folding and functional energy landscapes for adenylate kinase conformational change Enzyme function is often dependent on fluctuations between inactive and active structural ensembles. Adenylate kinase isolated from Escherichia coli (AK e ) is a small phosphotransfer enzyme in which interconversion between inactive (open) and active (closed) conformations is rate limiting for catalysis. AK e has a modular three-dimensional architecture with two flexible substrate-binding domains that interact with the substrates AMP, ADP and ATP. Here, we show by using a combination of biophysical and mutagenic approaches that the interconversion between open and closed states of the ATP-binding subdomain involves partial subdomain unfolding/refolding in an otherwise folded enzyme. These results provide a novel and, possibly general, molecular mechanism for the switch between open and closed conformations in AK e . Structural plasticity in proteins is intimately linked to their function. For example, the activity of many signal transducing enzymes is associated with large conformational changes between active and inactive states [1] , [2] . Moreover, many proteins undergo significant conformational changes on interaction with target proteins or small ligands [3] , [4] . In analogy to the energy landscape model of protein folding [5] , transitions between native conformational states in folded proteins are thought to be achieved through multiple pathways [6] , [7] . Qualitative descriptions of conformational changes can be inferred from analysis of the stable ground states. Hinge and shear motions, and combinations thereof, have been proposed to facilitate conformational changes [8] . What is not yet clear is the molecular mechanism, including information on transition states and other transient intermediates, of conformational change in the native states of proteins. It is difficult to probe intermediates and transition states involved in conformational changes, as these states are short lived and not directly accessible by spectroscopy. Here, we describe experiments that allow us to decipher the molecular mechanism of a large-scale conformational change in adenylate kinase (AK). AK catalyses the reversible phosphoryl transfer reaction Mg 2+ ATP+AMP↔Mg 2+ ADP+ADP and has the primary role of maintaining the energy balance in cells. The importance of AK is reflected in its ubiquitous presence in many different organisms and tissues [9] . AK isolated from E. coli (AK e ) uses a random bi–bi mechanism during catalysis [10] , [11] and the phosphoryl transfer chemistry likely follows an associative mechanism [12] . 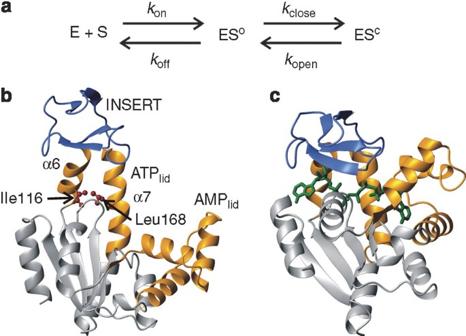Figure 1: Kinetic and structural models for substrate binding by AK. (a) Nucleotide binding mechanism for AK. E corresponds to enzyme, S to substrate, ESOto a transient substrate-bound encounter complex, ESCto the active conformation of AK. Superscripts 'O' and 'C' refer to AK in open (inactive) and closed (active) conformations. The rate constants for association and dissociation of ESOare given bykonandkoff, whereas the rate constants for conformational change are given bykcloseandkopen. (b,c) Structures of AKeduring the extreme stages of catalysis. ATPlid(residues 113–176) and AMPlid(residues 28–72) are coloured gold and the INSERT segment of the ATPlid(residues 122–15943) is coloured blue. (b) Substrate-free open AKe(4AKE.pdb). Residues isoleucine 116 and leucine168, which are mutated into glycine in this study, are highlighted with ball and stick representations, and the location of alpha helices, α6 and α7, is indicated. (c) Closed AKewith bound Ap5A (1AKE.pdb). All molecular graphic images in this report were prepared with MolMol44. A simplified nucleotide-binding mechanism for AK is shown in Figure 1 . Figure 1: Kinetic and structural models for substrate binding by AK. ( a ) Nucleotide binding mechanism for AK. E corresponds to enzyme, S to substrate, ES O to a transient substrate-bound encounter complex, ES C to the active conformation of AK. Superscripts 'O' and 'C' refer to AK in open (inactive) and closed (active) conformations. The rate constants for association and dissociation of ES O are given by k on and k off , whereas the rate constants for conformational change are given by k close and k open . ( b , c ) Structures of AK e during the extreme stages of catalysis. ATP lid (residues 113–176) and AMP lid (residues 28–72) are coloured gold and the INSERT segment of the ATP lid (residues 122–159 [43] ) is coloured blue. ( b ) Substrate-free open AK e ( 4AKE .pdb). Residues isoleucine 116 and leucine168, which are mutated into glycine in this study, are highlighted with ball and stick representations, and the location of alpha helices, α6 and α7, is indicated. ( c ) Closed AK e with bound Ap5A ( 1AKE .pdb). All molecular graphic images in this report were prepared with MolMol [44] . Full size image The structure of AK e has been solved in substrate-free (open) [13] and inhibitor P 1 ,P 5 –Di(adenosine-5′)pentaphosphate (Ap5A [14] )-bound (closed) conformations [15] ( Fig. 1 ). NMR experiments conducted in our laboratory have shown that the closed conformation represents the catalytically active state in which phosphoryl transfer occurs [16] . AK e is a modular enzyme and consists of a CORE subdomain and ATP- and AMP-binding subdomains ( Fig. 1 ). Both ATP and AMP subdomains (ATP lid and AMP lid ) undergo significant conformational changes in response to substrate binding. The large conformational change has at least two functional origins: first, the active site must be dehydrated to avoid non-productive hydrolysis of ATP and, second, the substrates are aligned optimally for the phosphoryl-transfer chemistry. The local thermodynamic stability of the nucleotide-binding subdomains is significantly lower compared with the CORE, and the subdomains fold and unfold in a non-cooperative manner [17] . From a functional perspective, this feature allows the rearrangement in backbone hydrogen bonding patterns (observed during the open-to-closed transition) without provoking global unfolding of the entire protein. It was recently reported that, at temperatures above 35 °C, the INSERT segment in ATP lid ( Fig. 1 ) selectively unfolded, resulting in reduced Ap5A-binding affinity [18] . The state with an unfolded INSERT segment was denoted as a 'binding incompetent state' and appears to be an intermediate on the global unfolding pathway. Selective unfolding of INSERT agrees with our previous observation that ATP lid can be selectively unfolded without perturbing the structure of other parts of the enzyme [17] . The structural plasticity of AK e is strongly coupled to its catalytic efficiency, as reopening of substrate binding domains with bound nucleotides is rate limiting for catalysis [19] . This observation is consistent with the finding that the rate-limiting step involves dissociation of bound nucleotides [10] . Notably, the conformational changes of ATP lid and AMP lid occur even in the absence of substrates [20] . Addition of ATP and AMP gradually shifts the conformational equilibrium towards the closed state [16] . Apparently, the conformational dynamics that is relevant for substrate binding is an intrinsic property of AK e . This feature of enzyme function has also been observed for dihydrofolate reductase [21] , cyclophilin A [22] and RNase A [23] . There exist two contradicting models for the open/closed conformational change of the nucleotide-binding subdomains in AK: (i) 'induced fit' and (ii) 'cracking' models. On the basis of an analysis of crystallographic structures, the induced fit model has been proposed for closure of both ATP lid and AMP lid . In this model, segments in between hinge regions are spatially translated as rigid bodies [24] . Closure of ATP lid is accomplished by rotation of the INSERT segment around helices α6 and α7, which in turn rotate around the CORE ( Fig. 1 ). In the 'cracking' model, significant strain energy is built up for residues in α6 and α7 during the reaction, and, at the transition state, this strain is released by a local unfolding event. At the downhill side of the activation energy barrier, the protein refolds and the thermodynamic minimum corresponding to the closed state is reached [25] , [26] . The cracking model was inferred from coarse-grained modelling and the principle of minimal frustration [26] . There are no experimental studies verifying which mechanism is used by AK. We previously identified a hydrophobic cluster in ATP lid that consists of isoleucine (Ile) 116, valine (Val) 117, Val 164 and leucine (Leu) 168. Simultaneous mutation of these positions to glycine selectively unfolded the entire ATP lid without perturbing the structures of the CORE and AMP lid subdomains [17] . Surprisingly, this variant is capable of binding the inhibitor Ap5A (unpublished results). The hydrophobic cluster constituted of these four residues is conserved in the AK family, as evident from a published sequence alignment of 250 AK sequences [27] . On the basis of our observations on the quadruple mutant, we have, in this study, designed single (Ile116Gly, 'M1') and double (Ile116Gly and Leu168Gly, 'M2') mutated variants of AK e in order to probe the reaction mechanism of ATP lid closure. Our data show that segments in ATP lid unfold and subsequently refold during the open-to-closed conformational transition, and show that folding and function are closely coupled events in AK e . Structure of mutated AK e in apo states The structures of M1 and M2 AK e variants were assessed with far-ultraviolet circular dichroism (CD) spectroscopy ( Supplementary Fig. S1 ). Wild-type (WT) AK e displays two distinct minima in the CD signal at 208 and 222 nm, in agreement with previous results [28] . Single and double mutations decrease the helical content of AK e , as inferred from a reduction in the intensity of CD signals at 208 and 220 nm. As discussed below, this effect is dependent on selective destabilization/unfolding of α6 and α7. A qualitative analysis of the CD spectra using CDNN software (copyright Dr Gerald Böhm) provided deconvoluted helical contents of 64, 54 and 39 (±5) % for WT, M1 and M2, respectively. The reduction of helical content in M2 compared with WT AK e is consistent with a complete loss of the helical structure of α6 and the section of α7 belonging to the ATP lid . Taking the helical contents of WT AK e and M2 as benchmarks for folded and unfolded α6 and α7, M1 is placed in between with a fraction of folded α6, α7 of ∼ 60%. 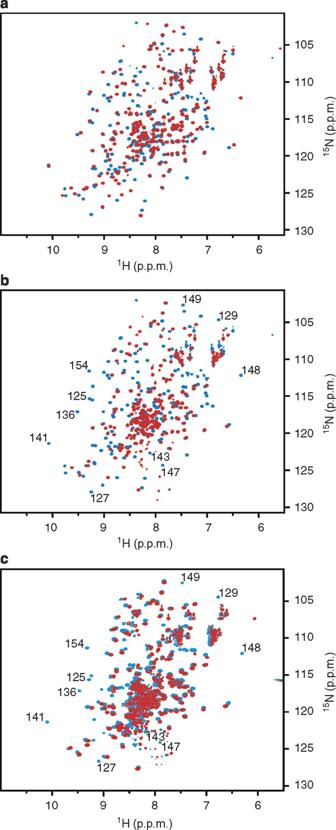Figure 2: NMR spectra of substrate-free WT AKe, M1 and M2 mutants. In (a) and (b), WT AKeis shown with blue contouring and the two mutants are contoured red. (a) Superimposition of1H-15N HSQC spectra of WT AKeand M1 acquired at 25 °C. (b) Superimposition of1H-15N HSQC spectra of WT AKeand M2 acquired at 25 °C. Selected resonances in the INSERT segment of the ATPlidthat are missing in the M2 mutant are indicated. (c) Superimposition of1H-15N HSQC spectra of M2 acquired at 25 °C (red contours) and 15 °C (blue contours). Selected resonances (same set as inb) corresponding to residues in the INSERT segment in ATPlidare indicated. 1 H- 15 N Heteronuclear Single-Quantum Coherence (HSQC) spectra of the two mutants superimposed on the WT are shown in Figure 2a,b . A visual inspection shows that M1 resembles the WT enzyme with many overlapping peaks distributed over the whole spectrum. In contrast, M2 shows marked spectral differences, compared with the WT enzyme. Figure 2: NMR spectra of substrate-free WT AK e , M1 and M2 mutants. In ( a ) and ( b ), WT AK e is shown with blue contouring and the two mutants are contoured red. ( a ) Superimposition of 1 H- 15 N HSQC spectra of WT AK e and M1 acquired at 25 °C. ( b ) Superimposition of 1 H- 15 N HSQC spectra of WT AK e and M2 acquired at 25 °C. Selected resonances in the INSERT segment of the ATP lid that are missing in the M2 mutant are indicated. ( c ) Superimposition of 1 H- 15 N HSQC spectra of M2 acquired at 25 °C (red contours) and 15 °C (blue contours). Selected resonances (same set as in b ) corresponding to residues in the INSERT segment in ATP lid are indicated. 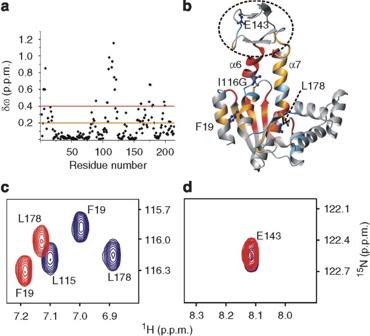Figure 3: Propagation of structural perturbations in the M1 mutant. Perturbations resulting from the mutation were quantified on the basis of combined absolute15N and1H chemical shift differences between WT and mutant, calculated according to δω=0.2 × |Δ15N|+|Δ1H| (p.p.m.)16. As a result of the point mutation, structural rearrangements are propagated throughout the entire ATPlid, with the exception of residues in the INSERT segment (indicated with a dashed oval). (a) Chemical shift differences for non-mutated residues plotted against the primary sequence; threshold values used in (b) are indicated with red and orange lines. (b) Chemical shift perturbations displayed on the open AKestructure (4AKE.pdb); perturbations are colour coded as follows: red δω>0.4 p.p.m., orange 0.4>δω>0.2 p.p.m.; residues that are unassigned in either WT or M1 and proline residues are coloured blue. The mutation site and residues F19, E143 and L178 are shown as dark blue ball and sticks. (c,d) Expansions of1H-15N HSQC spectra of WT (blue) and M1 (red) AKe. (c) Chemical shift perturbations of L178 and F19 (both 0.27 p.p.m., calculated as stated above); both these residues are accordingly coloured orange in (b). (d) The chemical shift of E143 is identical in the mutant and WT spectra, consistent with identical structures in the INSERT segment. Full size image Combined absolute differences in 1 H and 15 N chemical shifts between the M1 mutant and WT AK e are shown in Figure 3a, and these results are plotted on the open AK e structure in Figure 3b . Significant chemical shift differences are found in α6, α7, and these are propagated to a large part of the CORE. In light of the results from CD spectroscopy and from our previous analysis of a quadruple AK e mutant [17] , the chemical shift perturbations in α6 and α7 depend on a local unfolding event. The differences observed in the CORE are not dependent on unfolding, as we have shown that the quadruple mutant does not affect the topology of this domain [17] . The region of the CORE that shows shift changes ( Fig. 3b,c ) is part of a dense interaction network, and the observed changes may be reflecting minute changes in the packing of hydrophobic side chains. Interestingly, residues in the INSERT segment show no significant chemical shift perturbations in M1 ( Fig. 3d ), showing that this part of the molecule is structurally unaffected by the mutation. This result suggests that ATP lid is composed of two cooperatively folding units: the INSERT and α6, α7 parts. Figure 3: Propagation of structural perturbations in the M1 mutant. Perturbations resulting from the mutation were quantified on the basis of combined absolute 15 N and 1 H chemical shift differences between WT and mutant, calculated according to δω=0.2 × |Δ 15 N|+|Δ 1 H| (p.p.m.) [16] . As a result of the point mutation, structural rearrangements are propagated throughout the entire ATP lid , with the exception of residues in the INSERT segment (indicated with a dashed oval). ( a ) Chemical shift differences for non-mutated residues plotted against the primary sequence; threshold values used in ( b ) are indicated with red and orange lines. ( b ) Chemical shift perturbations displayed on the open AK e structure ( 4AKE .pdb); perturbations are colour coded as follows: red δω>0.4 p.p.m., orange 0.4>δω>0.2 p.p.m. ; residues that are unassigned in either WT or M1 and proline residues are coloured blue. The mutation site and residues F19, E143 and L178 are shown as dark blue ball and sticks. ( c , d ) Expansions of 1 H- 15 N HSQC spectra of WT (blue) and M1 (red) AK e . ( c ) Chemical shift perturbations of L178 and F19 (both 0.27 p.p.m., calculated as stated above); both these residues are accordingly coloured orange in ( b ). ( d ) The chemical shift of E143 is identical in the mutant and WT spectra, consistent with identical structures in the INSERT segment. Full size image Partial assignments were obtained for the M2 mutant. The resonances corresponding to the ATP lid could not be assigned because of unfolding of this subdomain. On the basis of spectral similarities with published NMR spectra of a quadruple mutant [17] , we conclude that M2 has an unfolded ATP lid subdomain (in agreement with the CD results). On the other hand, many residues in the CORE and AMP lid could be assigned. In a spectrum recorded at 15 °C, resonances corresponding to the INSERT segment appeared at resonance frequencies very close to that of WT at the same temperature ( Fig. 2c ). This result implies that the INSERT retains the WT structure at 15 °C and that the absence of these resonances at 25 °C is due to conformational fluctuations on the μs–ms time scale. Notably, resonances corresponding to α6 and α7 could not be observed at 15 °C. The decoupling between folding of α6, α7 and the INSERT is thus a conserved feature of both M1 and M2 variants. Protein stability was studied by measuring thermal stability, which provides melting points ( T m ) and enthalpies of unfolding (Δ H vH ) at T m . Unfolding curves for the three AK e variants ( Fig. 4 ) were fitted to a two-state unfolding transition according to Equation (3). Both mutated variants show a modest decrease in T m compared with the WT ( Supplementary Table S1 ); however, the Δ H vH is significantly lower for both mutants. The large enthalpic difference is consistent with an unfolded ATP lid for the mutants at T m . The small effect on T m in light of the large enthalpic differences between WT and mutants is explained with the thermal transition being dominated by the CORE subdomain. 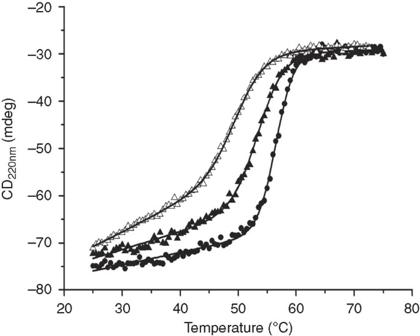Figure 4: Thermal denaturation of AKevariants. Unfolding was monitored with the CD signal at 220 nm for WT (filled circles), M1 (filled triangles) and M2 (open triangles). Solid lines represent nonlinear fits to Equation (3). Fitted parameters are summarized inSupplementary Table S1. Figure 4: Thermal denaturation of AK e variants. Unfolding was monitored with the CD signal at 220 nm for WT (filled circles), M1 (filled triangles) and M2 (open triangles). Solid lines represent nonlinear fits to Equation (3). Fitted parameters are summarized in Supplementary Table S1 . Full size image Local unfolding promotes ATP-binding affinity ATP-binding affinities and enthalpies between AK e variants and ATP were determined using isothermal titration calorimetry (ITC; Fig. 5 and Table 1 ). All experiments were performed in duplicate and the reported parameters are average values. Surprisingly, the binding affinities of the two mutants, M1 and M2, towards ATP are increased markedly compared with WT AK e . The observed dissociation constant ( K app d ) for WT is 51±13 μM (pH 7, 25 °C), with a calorimetric enthalpy (Δ H ITC ) of −2.2±0.4 kJ mol −1 . Binding between ATP and AK e has previously been quantified with other biophysical techniques [16] , [29] , [30] . These independent studies provided K app d values in the range of 35–53 μM in good agreement with our ITC data. As ATP binding is associated with a low enthalpy change and baseline distortions, we performed a control experiment using Ap5A ( Supplementary Fig. S2 ). Ap5A binds AK e with a K app d of 0.14±0.5 μM and a Δ H ITC of −19±5 kJ mol −1 , in good agreement with published results [18] . K app d values quantified for M1 and M2 are 0.78±0.2 and 0.98±0.3 μM, respectively. All AK variants bind to ATP with a one-to-one stoichiometry as evident by fitted n values ( Table 1 ), in agreement with previous NMR studies that showed one-to-one binding between WT AK e and ATP [16] . Notably, binding of ATP to M1and M2 is associated with significantly increased Δ H ITC , −51±2 and −110±10 kJ mol −1 , respectively. This difference is explained with a coupled folding and binding event in the case of M1 and M2, in which Δ H ITC is a cumulative sum of ATP lid folding (Δ H fol ) and ATP-binding enthalpies (Δ H bind ), according to Equation (1) ( f u refers to the degree of ATP lid unfolding). 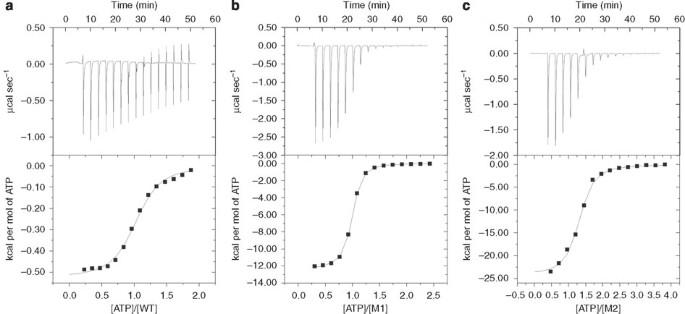Figure 5: Increased binding affinities towards ATP for mutated enzymes relative to WT AKe. Apparent dissociation constants and enthalpy on binding were measured using ITC. The baseline-corrected instrumental response is shown in the upper panels, and the integrated data (squares), together with the best fits (solid lines) according to a one-site binding model, are shown in the lower panels for (a) WT AKe, (b) M1 and (c) M2. Fitted parameters are summarized inTable 1. Figure 5: Increased binding affinities towards ATP for mutated enzymes relative to WT AK e . Apparent dissociation constants and enthalpy on binding were measured using ITC. The baseline-corrected instrumental response is shown in the upper panels, and the integrated data (squares), together with the best fits (solid lines) according to a one-site binding model, are shown in the lower panels for ( a ) WT AK e , ( b ) M1 and ( c ) M2. Fitted parameters are summarized in Table 1 . Full size image Table 1 ITC data for ATP binding to AK e variants at pH 7 and 25 °C Full size table The structural analysis showed that helices α6 and α7 are partially unfolded in M1 and M2; thus, Δ H ITC of ATP binding includes folding of these helices. The difference in calorimetric enthalpy for the two mutants scales with the degree of unfolding in ATP lid observed using CD and NMR spectroscopy. The entropic term is in favour of ATP binding in the case of WT AK e , presumably because of the release of solvent molecules hydrating both the substrate and the enzyme. In contrast, both M1 and M2 display strong enthalpy/entropy compensation for ATP binding. The large enthalpic components in M1 and M2 are paralleled with a significant entropic penalty. This may be explained by restriction of the main chain as a consequence of the coupled folding/binding event in the ATP lid in these mutants. Preservation of conformational dynamics in mutated AK e Chemical shifts can be used to distinguish between open and closed conformations of AK. WT AK e in complex with Ap5A mainly populates the closed conformation [16] . The 1 H- 15 N HSQC spectrum of M2, in complex with Ap5A ( Supplementary Fig. S3 ), is of high quality and closely resembles the spectrum of Ap5A-bound WT AK e [16] . Residues with significant chemical shift perturbations are localized to regions surrounding the sites of mutations ( Supplementary Fig. S4 ). The similarity between WT and M2 HSQC spectra is a strong indication that M2 is adopting a structure in complex with Ap5A that closely resembles the closed AK e conformation. Interestingly, most of the resonances that are missing (because of unfolding) in ATP lid in the M2 apo state are visible and assigned in the Ap5A complex. Apparently, M2 undergoes a coupled folding and binding event on interaction with Ap5A. To directly verify that M2 is populating a closed AK e conformation in complex with Ap5A, we made use of a chemical shift-based method previously developed in our laboratory [16] . There exists a strong linear correlation with a slope of close to unity when chemical shift perturbations between M2 and WT (both bound to Ap5A) are compared ( Supplementary Fig. S5 ). The linear correlation (with a slope near one) is evidence for a closed M2 conformation in complex with Ap5A, and enables the use of chemical shifts of M2 in complex with Ap5A as residue-specific markers of a fully closed enzyme. As α6 and α7 are unfolded to a degree in between M2 and WT, it is safe to assume that M1 populates a closed conformation in complex with Ap5A as well. The results show that M2 and M1 are functional enzymes that retain the ability to adopt the closed state. Structure of AK e :ATP complexes The structural response to ATP binding in M1 and M2 was addressed by quantifying chemical shift perturbations in protein samples saturated with ATP. The quantitative analysis is restricted to the M1 variant as assignments of the ATP lid are missing in M2. However, the 1 H- 15 N HSQC spectra of ATP-saturated M1 and M2 are very similar ( Supplementary Fig. S6 ), implying that the corresponding ATP complexes adopt similar structures. Notably, the number of observable resonances of M2 is significantly increased in the M2:ATP complex compared with the apo state (compare Fig. 2b and Supplementary Fig. S6 ), which is complementary evidence of a coupled folding/binding reaction, in agreement with the ITC data. In Supplementary Figures S7 and S8 , the chemical shift perturbations in response to ATP binding for M1 and WT AK e are summarized. The spatial locations of residues that are most strongly affected by ATP binding are very similar in both enzyme variants. Apparently, M1 binds to ATP with the same interaction surface as WT and as such is a functional enzyme with respect to ATP binding. This inference is valid for M2 as well, in light of the resemblance of M1 and M2 NMR spectra in ATP-saturated states. Mutations modulate the open-to-closed equilibrium constant We have previously shown that the ATP lid in AK e interconverts between open and closed conformations in the presence of bound ATP [16] . A detailed description of the method used to quantify populations is provided in the Supplementary Methods and in Supplementary Figures S9 , S10 . Equilibrium open and closed populations of both WT and the M2 variant in their ATP-bound states were determined by comparing chemical shifts in apo (open), Ap5A-bound (closed) and ATP-saturated states ( Fig. 6 ). As assignments of ATP lid in the M2 apo state was missing, the analysis was centred on the N- and C-terminal α-helices (inset Fig. 6a ). Both these α-helices respond structurally to ATP binding in concert with ATP lid and are valid markers of the open/closed equilibrium ( Supplementary Information Fig. S2 and Table S2 in Ådén and Wolf-Watz [16] ). For WT AK e , the population of closed ATP lid in the ATP complex is 0.6, in good agreement with previous analysis [16] . The fraction of closed ATP lid is significantly increased in the M2:ATP complex, and, within the experimental uncertainty, the closed population is near 1. Apparently, the conformational equilibrium for the open/closed transition in the presence of ATP is strongly skewed towards the closed state as a consequence of the structural perturbation. As the NMR spectra of the ATP-saturated M1 and M2 variants are very similar, it appears likely that a similar shift in the open/closed equilibrium is valid for M1 as well. 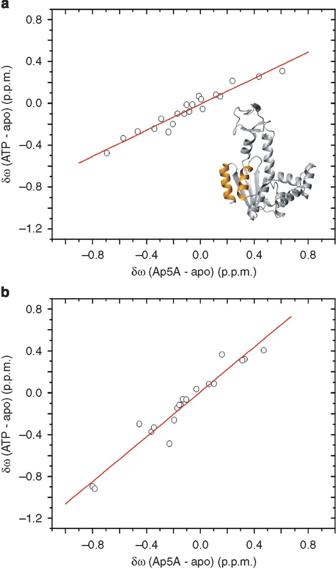Figure 6: Shift of open/closed equilibrium in ATP-saturated M2 versus WT AKe. Normalized chemical shift perturbations in ATP- and Ap5A-bound states referenced to the apo states are calculated according to δω=0.2Δ15N+Δ1H (p.p.m.). (a) Correlation between ATP and Ap5A chemical shift perturbations for WT AKe. The best-fitted straight line (red) has a slope of 0.62±0.07 with anRcoefficient of 0.97. In all, 20 residues were used in the analysis. Inset: positions of the residues analysed in WT and M2 are coloured gold on the open AKestructure. (b) Correlation between ATP and Ap5A chemical shift perturbations for the M2 variant. The best-fitted straight line (red) has a slope of 1.07±0.1 with anRcoefficient of 0.97; 19 residues were used in the analysis. Figure 6: Shift of open/closed equilibrium in ATP-saturated M2 versus WT AK e . Normalized chemical shift perturbations in ATP- and Ap5A-bound states referenced to the apo states are calculated according to δω=0.2Δ 15 N+Δ 1 H (p.p.m.). ( a ) Correlation between ATP and Ap5A chemical shift perturbations for WT AK e . The best-fitted straight line (red) has a slope of 0.62±0.07 with an R coefficient of 0.97. In all, 20 residues were used in the analysis. Inset: positions of the residues analysed in WT and M2 are coloured gold on the open AK e structure. ( b ) Correlation between ATP and Ap5A chemical shift perturbations for the M2 variant. The best-fitted straight line (red) has a slope of 1.07±0.1 with an R coefficient of 0.97; 19 residues were used in the analysis. Full size image Catalytic activities of AK e variants As product release is rate limiting for AK e catalysis [10] , [19] , the increased ATP-binding affinities of the M1 and M2 mutants are expected to hamper catalytic activities. Kinetic parameters with ATP as the variable and AMP as the constant substrate were quantified for M1, M2 and compared with that of WT AK e ( Table 2 ). As expected, k cat values were significantly reduced ( ∼ 40-fold) for the two mutants, and the reduction in k cat was very close to the (50-fold) increase in ATP-binding affinity. In addition, the increased ATP-binding affinities were reflected in decreased K ATP M values for the two mutants. Table 2 Kinetic parameters for AK e catalysis with ATP as variable substrate at 25 °C Full size table The two AK e variants studied here have segmentally disordered ATP lid domains at 25 °C. We have previously proposed that the entire ATP lid functions as one cooperatively folding unit [17] . In this study, we identified additional layers in complexity in the folding behaviour of ATP lid , namely, that α6 and α7 forms one folding unit and the INSERT segment forms a second. The mutated variants have significantly reduced vant't Hoff enthalpies of thermal unfolding but with only modest reduction in T m . This small perturbation in T m is a consequence of the weak thermodynamic coupling between ATP lid and CORE subdomains. From a functional perspective (in terms of ATP binding), the mutated variants display WT-like properties. First, the chemical shift perturbation patterns inflicted by ATP binding are strikingly similar to the WT, showing that the same interaction surface is used for ATP interaction in mutated and WT AK e . Second, both mutated variants can populate fully closed conformations in complex with the inhibitor Ap5A; thus, the enzymes retain the ability to close its substrate-binding motifs. As a consequence of the coupled folding/binding equilibrium in the M1 and M2 variant, the enthalpic contribution for ATP binding is significantly larger compared with that of WT AKe because of the cumulative effects of folding and binding enthalpies. The decreased enthalpies of ATP binding (favouring binding) are accompanied by increased entropic components (disfavouring binding) in the mutants. Such enthalpy/entropy compensation has been observed in other proteins that mechanistically utilize coupled folding/binding reactions to interact with substrates [31] . It is remarkable that structural mutations that destabilize the ATP lid are paralleled with an ∼ 50-fold increase in ATP-binding affinity. To identify the underlying molecular explanation, we analysed the formal expression for K app d following Figure 1a and obtained Equation (2) (see Supplementary Methods for derivation). In Equation (2), K d is the dissociation constant and K conf is the equilibrium constant for the open-to-closed equilibrium in the presence of bound ATP ( Supplementary Equation S4 ). An inspection of Equation (2) shows that the decreased K app d can originate from reduced K d or increased K conf values, relative to WT AK e . It is unlikely that K d is decreased in the mutants, as the structure of ATP lid is perturbed in both M1 and M2. On the other hand, the equilibrium constant for the open–closed transition ( K conf ) in the presence of bound ATP is significantly skewed in the M2 variant compared with WT AK e . In WT AK e and the M2 variant, the experimentally determined values of fractions closed ATP lid are 0.62±0.07 and 1.07±0.1, respectively. Assuming that K d adopts equal values in WT, M1 and M2, and with a WT K conf of 1.5 (0.6/0.4), Equation (2) was used to calculate a value of K conf equal to 124 that accounts for the observed reduction in K app d (from ∼ 50 μM in WT to ∼ 1.0 μM in the mutants). This value translates to fractions of open and closed conformations of around 0 and 1, respectively, in excellent agreement with our experimental observations. Apparently, the increased affinity for ATP in the mutant AK e variants is fully explained by a large shift in the open-to-closed equilibrium constant. If, on the other hand, mutations would stabilize a 'binding incompetent state', that is, a disordered ATP lid on a reaction pathway towards global protein unfolding, the observed binding affinity would decrease ( Supplementary Equation S6 ). As the ATP-binding affinity is increased as a result of the ATP lid destabilization, our mutations modulate the native free-energy landscape on the reaction trajectory for subdomain closure. The effect of the mutations is to redistribute states that are present in WT AK e . It might seem intuitive that the chemical shifts of the mutant AK e variants should fall in between the chemical shifts of open and closed WT AK e . However, a detailed consideration of chemical shifts ( Supplementary Note and Supplementary Fig. S11 ) shows that this correlation is not expected. In good agreement with our model for catalysis (that is, rate-limiting dissociation of bound nucleotides), the M1 and M2 variants display ∼ 40-fold decrease in catalytic efficiency compared with WT AK e . The fact that mutations redistribute already existing states is in agreement with arguments discussed previously [7] . On the basis of these arguments, we propose that local disordering of α6 and α7 is part of the reaction trajectory for closure of the ATP lid ( Fig. 7 ). As both the stable ground states (open and closed) contain well-folded α6 and α7 helices, the conformational change follows an order-disorder-order mechanism, in agreement with the cracking model [25] , [26] . To the best of our knowledge, this is the first experimental observation of such a mechanism. The energetic prerequisite for our mechanistic model is that the local thermodynamic stability of α6 and α7, is sufficiently low to accommodate an unfolding/folding reaction. This boundary condition has been observed for AK isolated from three different organisms [17] , [32] . Thus, the energetic prerequisite for our model is generally met in the AK fold. The low structural stabilities in these key regions are also reflected in high B-factors in the substrate-free AK e structure [13] , [17] . Both residues mutated here (Ile 116 and Leu 168) are strongly conserved within the AK family [27] . In fact, the entire hydrophobic cluster (positions 116, 117, 164 and 168) in ATP lid identified by us previously [17] is conserved with a consensus sequence equivalent to the AK e sequence. In our proposed model, disruption of this cluster is part of the mechanism for ATP binding and, given the strong sequence conservation, the mechanism is likely to be general in the AK family. Protein folding is usually described using funnel-shaped energy landscapes [5] in which the native state exhibits minimal frustration [33] ; our results with an unfolding/folding reaction during a functional transition point towards an overlap between folding and functional energy landscapes. It is possible that the novel mechanism used by AK e during the open-to-close transition is also used by other proteins that undergo conformational changes. 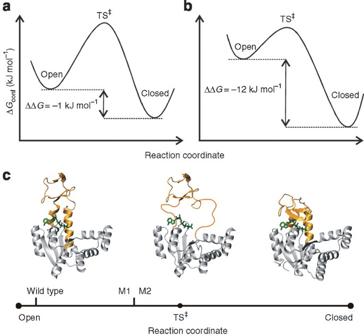Figure 7: Model for ATPlidclosure in AKe. Relative free-energy differences between open and closed ATPlidconformations in the presence of saturating ATP concentration for WT (a) and the M2 variant (b). The relative change in free energy (ΔΔGconf) is calculated fromKconfvalues of 1.5 and 124 (124 equals the minimum value that accounts for the increased ATP-binding affinity in M1 and M2 compared with WT) for WT and the M2 variant. Theyaxis in (a) and (b) is set arbitrarily such that the absolute values of the free energy for open, closed and transition state (TS‡) structures may in fact differ for the two enzymes. (c) Structural model of the conformational change in the ATPlidin the presence of bound ATP. The ATP complex is represented with yeast AKein complex with the non-hydrolysable ATP analogue AMPPCF2P45. The structures going from open to partially unfolded to closed are arranged as a function of the reaction coordinate. The relative positions of the WT and the M1, M2 variants are indicated on the reaction coordinate and should be interpreted as a qualitative measure of the distance to the transition state. Figure 7: Model for ATP lid closure in AK e . Relative free-energy differences between open and closed ATP lid conformations in the presence of saturating ATP concentration for WT ( a ) and the M2 variant ( b ). The relative change in free energy (ΔΔ G conf ) is calculated from K conf values of 1.5 and 124 (124 equals the minimum value that accounts for the increased ATP-binding affinity in M1 and M2 compared with WT) for WT and the M2 variant. The y axis in ( a ) and ( b ) is set arbitrarily such that the absolute values of the free energy for open, closed and transition state (TS ‡ ) structures may in fact differ for the two enzymes. ( c ) Structural model of the conformational change in the ATP lid in the presence of bound ATP. The ATP complex is represented with yeast AK e in complex with the non-hydrolysable ATP analogue AMPPCF 2 P [45] . The structures going from open to partially unfolded to closed are arranged as a function of the reaction coordinate. The relative positions of the WT and the M1, M2 variants are indicated on the reaction coordinate and should be interpreted as a qualitative measure of the distance to the transition state. Full size image A subpart of the mechanism identified for the conformational change in AK e , that is, disorder–order transitions, has been found in interactions between proteins and a diverse set of substrates. Disorder–order mechanisms coupled to substrate binding have been observed, for instance, in protein–DNA [34] , enzyme–substrate [31] , [35] , protein–peptide [36] and protein–protein [37] interactions. The folding of small proteins into a well-defined and compact active state is most often a highly cooperative process [38] without a significant population of non-native states. In a recent study, it was suggested that the cooperativity of the folding reaction is the result of natural selection [39] . It is intriguing that AK e uses cooperative unfolding/refolding to accommodate a large-scale conformational change during catalysis. An appealing hypothesis is that nature has made use of cooperative unfolding/refolding to add functional properties (such as conformational plasticity) to proteins. Protein preparation All AK e variants were prepared as described previously [19] . The concentrations of all proteins were determined using an extinction coefficient at 280 nm of 10.000 M −1 cm −1 . Site-specific mutagenesis Primer sequences for the M1 and M2 mutants were ordered from CyberGene. PCR-amplified DNA sequences encoding the mutant proteins were subcloned into the expression vector pET-3a (Novagen) using restriction enzymes Nde 1 and Bam HI. The final constructs were verified using DNA sequencing (Eurofins MWG Operon). Kinetic assays Enzyme kinetic parameters for ATP turnover in the direction of ADP formation were quantified at 25 °C using a coupled spectroscopic assay [10] . The ATP concentration was varied and the AMP concentration was fixed at 0.5 mM. NMR spectroscopy All NMR experiments were recorded on samples containing 0.7–1.2 mM 15 N-labelled proteins in 50 mM NaCl and 30 mM MOPS at pH 7.0 with 10% (v/v) 2 H 2 O. NMR experiments were carried out on a Bruker DRX 600 MHz spectrometer equipped with a 5-mm triple resonance z -gradient cryoprobe. The temperature was calibrated using an external probe inserted into the sample compartment of the NMR probe. Backbone resonance assignment of apo and substrate-saturated M1 and M2 mutants was obtained with 15 N nuclear overhauser effect spectroscopy-HSQC and HNHA experiments [40] . ATP and Ap5A (Sigma-Aldrich)-saturated enzymes were obtained by adding 20- and 2-mM substrate to protein samples, respectively. NMRPipe software [41] and ANSIG for Windows [42] were used for NMR data processing and visualization of spectra, respectively. ITC ITC experiments were carried out at 25 °C using an iTC200 Microcalorimeter (Microcal). The reference cell was filled with sample buffer, and protein-containing solutions were filled in the sample cell (200 μl volume) and titrated with ATP (40 μl). Substrate solutions were prepared in buffer (same batch) from the final step of protein purification (that is, gel filtration). Protein concentrations were 1.5 mM and 40 μM for WT titrations with ATP and Ap5A, respectively. M1 and M2 were at 20 μM for ATP titrations. The substrate concentration in the injection syringe was 10 times higher than the concentration of protein. A typical experiment consisted of an initial control injection of 1 μl, followed by 16 injections, each of 2.5 μl and 5 s duration, with a 180 s interval in between. ITC measurements were routinely taken in 50 mM NaCl and 30 mM MOPS at pH 7.0. In control experiments, the ligand (ATP) was injected into the buffer. Raw data were collected, corrected for ligand heats of dilution and integrated using the Microcal Origin software supplied with the instrument. A single-site binding model was fit to the data by a nonlinear regression analysis to yield binding constants ( K d ), observed enthalpies of binding (Δ H ITC ) and stoichiometry of binding ( n ). CD spectroscopy Far-ultraviolet CD spectra (190–260 nm, 25 °C, 1-mm path length) and temperature scans (15–85 °C at 222 nm, 0.1-mm path length) were collected in 10 mM Na-phosphate and 50 mM NaCl (pH 7.0) on a Jasco J-810 Spectropolarimeter. Thermal denaturation curves were fitted to Equation (3) assuming a two-state reaction. The reversibility of the thermal transitions was larger than 80%. Protein concentrations in CD experiments ranged between 5 and 10 μM. Where Here, S obs is the temperature-dependent spectroscopic signal, m f , m u and S f , S u are the slopes and intercepts of the folded and unfolded baselines, respectively, T is the absolute temperature, T m is the melting point, K u is the unfolding equilibrium constant and Δ H vH is the van't Hoff enthalpy of unfolding at T m . How to cite this article: Olsson, U. & Wolf-Watz, M. Overlap between folding and functional energy landscapes for adenylate kinase conformational change. Nat. Commun. 1:111 doi: 10.1038/ncomms1106 (2010).